Chromatin remodelling complex dosage modulates transcription factor function in heart development Dominant mutations in cardiac transcription factor genes cause human inherited congenital heart defects (CHDs); however, their molecular basis is not understood. Interactions between transcription factors and the Brg1/Brm-associated factor (BAF) chromatin remodelling complex suggest potential mechanisms; however, the role of BAF complexes in cardiogenesis is not known. In this study, we show that dosage of Brg1 is critical for mouse and zebrafish cardiogenesis. Disrupting the balance between Brg1 and disease-causing cardiac transcription factors, including Tbx5, Tbx20 and Nkx2–5, causes severe cardiac anomalies, revealing an essential allelic balance between Brg1 and these cardiac transcription factor genes. This suggests that the relative levels of transcription factors and BAF complexes are important for heart development, which is supported by reduced occupancy of Brg1 at cardiac gene promoters in Tbx5 haploinsufficient hearts. Our results reveal complex dosage-sensitive interdependence between transcription factors and BAF complexes, providing a potential mechanism underlying transcription factor haploinsufficiency, with implications for multigenic inheritance of CHDs. The transcriptional regulation of organogenesis has been well studied, and in the developing heart, combinatorial interactions between transcription factors are key to robust gene regulation [1] , [2] . Importantly, disease-causing mutations in several cardiac transcription factors are the underlying cause of human congenital heart defects (CHDs) [2] , [3] . Most of these mutations are predicted to cause haploinsufficiency; however, the mechanistic basis for the aberrant gene expression that results from reduced transcription factor dosage is not known. Mutations in cardiac transcription factor genes, such as TBX5 , NKX2–5 and GATA4 , all cause dominant inherited human CHD. These factors physically interact with each other, providing an effective mechanism for specific target activation and a potential explanation for their common disease-related haploinsufficiency [4] , [5] , [6] . Tbx5, Nkx2–5 and Gata4 also interact with the Swi/Snf-like Brg1/Brm-associated factors (BAF) chromatin remodelling complexes, in part via Baf60c, a cardiac-enriched subunit of the BAF complexes [7] . This interaction is key for the de novo induction of cardiac differentiation from embryonic mesoderm [8] , and depletion of Baf60c function leads to impaired heart development [7] . Identification of Baf60c and other BAF complex subunits that co-assemble to form cell-type-specific complexes has revealed the importance of BAF complexes as instructive factors in differentiation, rather than simply as chromatin-unwinding machines [7] , [9] , [10] , [11] . These specific BAF complexes perform discrete functions related to lineage specification and precursor differentiation. However, little is known about dosage sensitivity of tissue-specific BAF complexes or their links to DNA-binding transcription factors that are involved in similar processes. Mammalian BAF complexes include one of the two ATPases, Brm or Brg1 (ref. 10 ). Brm is dispensible for development, whereas Brg1 (also known as Smarca4) is absolutely essential for broad aspects of development in early mouse embryogenesis [12] , [13] . Thus, disrupting the function of Brg1 provides insights into the global function of BAF complexes during development. In the present study, we examined the role of Brg1 in heart development in mouse and zebrafish and tested its potential role in modulating the function of disease-related cardiac transcription factors. Our results reveal a dosage-sensitive interdependence between transcription factors and BAF complexes that modulates several aspects of heart formation. We conclude that the disruption of a delicate balance between CHD-causing transcription factors and BAF complexes is likely to be a mechanistic cause of CHDs because of transcription factor haploinsufficiency. Brg1 is critical for mouse heart development To assess the importance of Brg1 in the developing mammalian heart, we deleted Brg1 in developing ventricular myocytes, with a loxP-flanked Brg1 allele (referred to here as Brg1 f ) [14] and Nkx2.5::Cre , which is expressed mainly in ventricular myocytes from E8.5 onwards, with rare sporadic activity in endocardial cells [15] , [16] ( Fig. 1a and Supplementary Fig. S1 ). This Brg1 deletion led to highly variable defects in heart formation ( Fig. 1b,c ), perhaps partly because of variable and incomplete activity of the Cre-expressing transgene ( Fig. 1a and Supplementary Fig. S1 ). Most embryos did not survive past E10.5; however, a few (two pups from over ten litters) Nkx2.5::Cre ; Brg1 f/f mice were born alive. Severely affected embryos had a loss of normal ventricular chamber morphology ( Fig. 1b ), whereas the least severely affected, which survived to birth, had dilated disorganized ventricles, ventricular septation defects and a double outlet right ventricle ( Fig. 1c ). Most embryos had reduced chamber size and impaired looping ( Fig. 1d ). Expression of several cardiac genes was defective in Nkx2.5::Cre ; Brg1 f/f embryos ( Fig. 1d ), including Nppa (a marker of chamber myocardium), Tbx5 (a transcription factor that regulates Nppa ) and the trabecular growth factor Bmp10 . Reduced Bmp10 expression has also been shown in the deletion of Brg1 using Sm22a::Cre , and has been determined to be a critical downstream effector of Brg1-dependent gene regulation [17] . Our deletion using Nkx2.5::Cre , although variable in its effect, uncovers a broader Brg1-dependent programme of gene expression than that observed with Sm22a::Cre , most likely because of the earlier expression of Nkx2.5::Cre . Other cardiac genes, such as Nkx2–5 and Actc1, were expressed normally ( Fig. 1d ), indicating deregulation of a specific programme in Nkx2–5::Cre ; Brg1 f/f hearts. 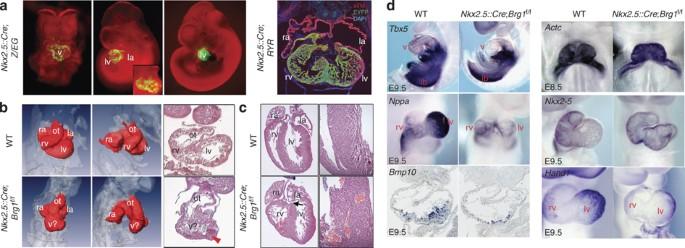Figure 1:Brg1is required for early mouse heart formation. (a) Activity of theNkx2.5::Cretransgene, using the Z/EG or RYR reporter, at E8.5, 9.5, 11 and 12.5. Inset for E9.5 embryo shows a ventral four-chamber view. For whole-mount pictures, green signal is the activity of the Z/EG reporter, whereas red signal is the bright-field illumination through a red filter. For the RYR reporter, a cryosection stained for anti-EYFP (green), alpha-tropomyosin (red) and 4,6-diamidino-2-phenylindole (blue) is shown. Original magnification: ×25 (whole-mount pictures), ×100 (sections). (b) Frontal view of OPT reconstructions (left panels), lateral view of OPT reconstructions (middle panels) and histology (rightmost panels) of WT andBrg1mutant (Nkx2.5::Cre;Brg1f/f) mice at E9.5. Arrowhead shows thickened ventricular wall. (c) Histology of postnatal day (P) 1 hearts. Arrow shows membranous ventricular septal defect and double outlet right ventricle in theNkx2.5::Cre;Brg1f/fheart. Close-up of the interventricular septum (right panels) shows disorganized septum formation. Original magnification: ×100. (d) Gene expression in WT andNkx2.5::Cre;Brg1f/fmice at E8.5 (Actc1) or E9.5 (all other genes) shows decreasedTbx5,Nppa, Bmp10andHand1expression. la, left atrium; lb, limb bud; lv, left ventricle; ra, right atrium; rv, right ventricle; v, ventricle; v?, ventricle of ambiguous identity. Figure 1: Brg1 is required for early mouse heart formation. ( a ) Activity of the Nkx2.5::Cre transgene, using the Z/EG or RYR reporter, at E8.5, 9.5, 11 and 12.5. Inset for E9.5 embryo shows a ventral four-chamber view. For whole-mount pictures, green signal is the activity of the Z/EG reporter, whereas red signal is the bright-field illumination through a red filter. For the RYR reporter, a cryosection stained for anti-EYFP (green), alpha-tropomyosin (red) and 4,6-diamidino-2-phenylindole (blue) is shown. Original magnification: ×25 (whole-mount pictures), ×100 (sections). ( b ) Frontal view of OPT reconstructions (left panels), lateral view of OPT reconstructions (middle panels) and histology (rightmost panels) of WT and Brg1 mutant ( Nkx2.5::Cre;Brg1 f / f ) mice at E9.5. Arrowhead shows thickened ventricular wall. ( c ) Histology of postnatal day (P) 1 hearts. Arrow shows membranous ventricular septal defect and double outlet right ventricle in the Nkx2.5::Cre;Brg1 f / f heart. Close-up of the interventricular septum (right panels) shows disorganized septum formation. Original magnification: ×100. ( d ) Gene expression in WT and Nkx2.5::Cre;Brg1 f / f mice at E8.5 ( Actc1 ) or E9.5 (all other genes) shows decreased Tbx5 , Nppa, Bmp10 and Hand1 expression. la, left atrium; lb, limb bud; lv, left ventricle; ra, right atrium; rv, right ventricle; v, ventricle; v?, ventricle of ambiguous identity. Full size image We conclude that Brg1 regulates specific programmes of gene expression in the developing heart that are critical for differentiation of cardiac myocytes and cardiac morphogenesis. Brg1 is critical for zebrafish heart development The BAF complex is conserved throughout evolution [10] . Zebrafishes have a single BAF complex ATPase, brg1 . young , a loss-of-function mutation of brg1 (refs 18 , 19 ), results in defects in retinal neurogenesis and pericardial oedema, which often indicates a defective heart function. We isolated a new mutation in brg1 , brg1 s481 , which is predicted to be a null allele ( Supplementary Fig. S2 ); this mutation creates a premature stop codon, predicting a truncation at amino-acid residue 252 (of 1,627), deleting all functional domains including the ATPase/SNF2 domain and the bromodomains. This mutation fails to complement the published yng allele [18] , [19] and is phenocopied by morpholino oligonucleotide (MO) treatment (see below), consistent with a null allele. These mutants formed a heart; however, after 48 h of development, the heart became hypoplastic and had severe arrhythmias with sporadic arrests in contraction ( Fig. 2a,b ; Supplementary Movies 1 and 2 ). The survival of brg1 mutant embryos to a late stage is likely related to the presence of maternal brg1 transcripts [19] . To knock down brg1 in other transgenic lines, translation-inhibiting MOs [20] were injected. Knockdown of brg1 by MO does not alter endocardial differentiation, and vascular development occurred normally ( Supplementary Fig. S3 ). However, the heart chamber displayed severe stenosis ( Fig. 2c,d ). Co-injection of an MO targeting p53 was used to investigate a role for cell death in the brg1 cardiac phenotype [21] . Injection of p53 MO into brg1 mutant embryos resulted in an identical cardiac phenotype to that observed in uninjected mutant siblings ( Supplementary Fig. S3 ). Gene expression analysis ( Fig. 2e ) demonstrated that, although differentiation of both heart chambers occurred properly, brg1 s481 zebrafish had lost the regionalization of nppa expression, which marks 'working' myocardium in fish and mice [22] ; this is reminiscent of the loss of Brg1 in the mouse. Expression of atrioventricular canal-specific genes, including bmp4 , tbx2b and notch1b , was abnormal in brg1 s481 embryos, suggesting patterning abnormalities in brg1 mutant zebrafish embryos. Expression of the Na + /Ca ++ exchanger ( Ncx ) was elevated in brg1 s481 embryos, which could explain contractility defects in brg1 s481 embryos [23] , [24] . We conclude that, in zebrafish, as in the mouse, brg1 is required for a specific programme essential for cardiac morphogenesis and patterning. 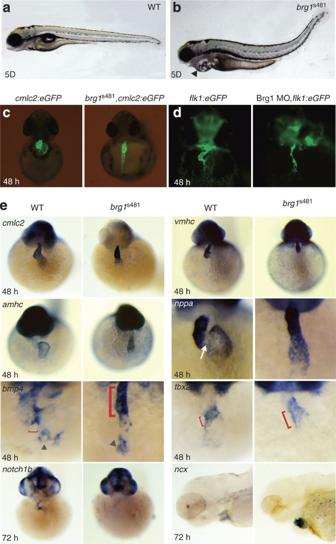Figure 2: Loss of Brg1 leads to heart development defects in the zebrafish embryos. (a,b) Lateral views at 5 dpf of WT (a) andbrg1s481(b) zebrafish embryos. Arrowhead inbshows pericardial oedema. (c,d) Frontal views of WT orbrg1s481zebrafish embryos at 48 hpf, showing myocardium, labelled withcmlc2:eGFP(c), and endocardium, labelled withflk1:eGFP(d). Original magnification: ×100. (e) Cardiac gene expression in WT andbrg1s481zebrafish embryos for indicated transcripts (left panels, top to bottom:cmlc2,amhc,bmp4andnotch1b; right panels, top to bottom:vmhc,nppa,tbx2bandncx). White arrow shows normal absence ofnppaat the atrioventricular (AV) junction, grey triangles show staining of pacemaker cells, red brackets show normal and expanded domains of AV canal markers (bmp4andtbx2b). Original magnification: ×200. Figure 2: Loss of Brg1 leads to heart development defects in the zebrafish embryos. ( a , b ) Lateral views at 5 dpf of WT ( a ) and brg1 s481 ( b ) zebrafish embryos. Arrowhead in b shows pericardial oedema. ( c , d ) Frontal views of WT or brg1 s481 zebrafish embryos at 48 hpf, showing myocardium, labelled with cmlc2:eGFP ( c ), and endocardium, labelled with flk1:eGFP ( d ). Original magnification: ×100. ( e ) Cardiac gene expression in WT and brg1 s481 zebrafish embryos for indicated transcripts (left panels, top to bottom: cmlc2 , amhc , bmp4 and notch1b ; right panels, top to bottom: vmhc , nppa , tbx2b and ncx ). White arrow shows normal absence of nppa at the atrioventricular (AV) junction, grey triangles show staining of pacemaker cells, red brackets show normal and expanded domains of AV canal markers ( bmp4 and tbx2b ). Original magnification: ×200. Full size image To uncover the cellular mechanisms underlying loss of brg1 in zebrafish, cardiomyocyte migration, proliferation and shape were analysed. During cardiac cone tilting, an early event in the formation of the zebrafish heart tube, atrial myocardium undergoes left-directed anterior migration [25] ( Fig. 3a–c ; Supplementary Movie 2 ). In brg1 morphants, anterior cardiomyocytes, especially those on the right side of the heart, displayed randomized trajectories ( Fig. 3d–f ; Supplementary Movie 3 ), resulting in the failure of proper heart jogging, which is indispensable for subsequent heart looping and chamber formation. We monitored the growth of the heart by counting the number of cardiomyocytes at different time points ( Fig. 3g–n ). At early stages, cell numbers between control and brg1 morphants were comparable (at 28 hpf, 166±12 ( n =4) cardiomyocytes in wild type (WT) hearts versus 145±14 in brg1 morphants ( n =5)). As development proceeded, however, growth in myocardial cell number obviously lagged in brg1 morphants and appeared to halt by 48 hpf (251±13 ( n =6) in WT hearts versus 173±14 in brg1 morphants ( n =4); Fig. 3o ; Supplementary Movies 4 and 5 ). 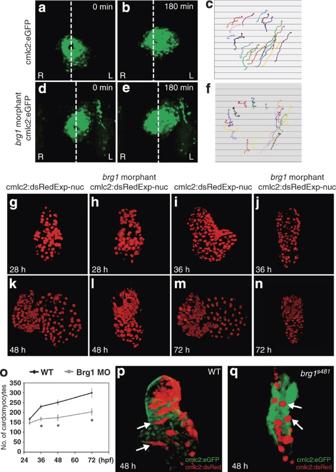Figure 3: Defective cardiomyocyte migration and cell shape in zebrafishbrg1mutants. (a–f) Imaging of atrial cell migration in WT embryos (a–c) andbrg1morphants (d–f). (a,b,d,e) Dorsal views of heart in Tg(cmlc2:eGFPtwu34) embryos between 18 and 21 hpf; dotted white lines indicate the embryonic midline. (c,f) Arrows of different colours indicate the trajectories of individual cells. Original magnification: ×200. (g–o) Measurement of cardiomyocyte numbers. Three-dimensional reconstructions of the nuclear DsRed signal fromTg(cmlc2:dsRedExp-nuchsc4) embryos are shown (g–n). The 28 hpf embryos (g, h) are shown in dorsal view, the 36 hpf (i,j), 48 hpf (k,l) and 72 hpf (m,n) embryos are shown in anterior views. (o) Quantitation of cardiomyocyte cell numbers. Data are mean±s.d.,n=5–8 embryos; *P<0.05 byt-test. Original magnification: ×400. (p,q) Three-dimensional assessment of cell morphologies in Tg(cmlc2:eGFPtwu34)-expressing hearts that exhibit mosaic expression of Tg(cmlc2:dsRedExp-nuchsc4). Arrows point to representative cells. (p) WT cells transplanted; (q)brg1s481cells transplanted. Original magnification: ×400. A, atrium; L, left; R, right; V, ventricle. Figure 3: Defective cardiomyocyte migration and cell shape in zebrafish brg1 mutants. ( a – f ) Imaging of atrial cell migration in WT embryos ( a – c ) and brg1 morphants ( d – f ). ( a , b , d , e ) Dorsal views of heart in Tg( cmlc2:eGFP twu34 ) embryos between 18 and 21 hpf; dotted white lines indicate the embryonic midline. ( c , f ) Arrows of different colours indicate the trajectories of individual cells. Original magnification: ×200. ( g – o ) Measurement of cardiomyocyte numbers. Three-dimensional reconstructions of the nuclear DsRed signal from Tg(cmlc2:dsRedExp-nuc hsc4 ) embryos are shown ( g – n ). The 28 hpf embryos ( g, h ) are shown in dorsal view, the 36 hpf ( i , j ), 48 hpf ( k , l ) and 72 hpf ( m , n ) embryos are shown in anterior views. ( o ) Quantitation of cardiomyocyte cell numbers. Data are mean±s.d., n =5–8 embryos; * P <0.05 by t -test. Original magnification: ×400. ( p , q ) Three-dimensional assessment of cell morphologies in Tg( cmlc2:eGFP twu34 )-expressing hearts that exhibit mosaic expression of Tg( cmlc2:dsRedExp-nuc hsc4 ). Arrows point to representative cells. ( p ) WT cells transplanted; ( q ) brg1 s481 cells transplanted. Original magnification: ×400. A, atrium; L, left; R, right; V, ventricle. Full size image During zebrafish heart development, confined myocardial cell-shape changes are a key parameter in cardiac morphogenesis [22] . In WT embryos, outer curvature cardiomyocytes became flattened and elongated and were aligned relative to each other ( Fig. 3p ; Supplementary Movie 6 ). In brg1 s481 embryos, cardiomyocytes had a cuboidal shape throughout the heart ( Fig. 3q ; Supplementary Movie 7 ). Because of the altered and variable cell shape, it is difficult to assess cell size, and thus we have not quantified this parameter; however, cell size did not appear to be grossly altered. As the changes in cell shape require a balance between extrinsic (blood flow) and intrinsic (contractility) biomechanical forces [22] , we examined the circulation in brg1 s481 embryo ( Supplementary Movie 8 ). The circulation in mutant embryos was slower than that in WT embryos at 36 hpf, but still robust, suggesting that reduced circulation did not cause the abnormal myocyte shapes. Rather, the cell-shape changes in brg1 mutants may reflect either an intrinsic defect in myocardial morphogenesis and/or be secondary to abnormal heart contractility. CHDs in Brg1 haploinsufficient mice The defects upon cardiac-specific deletion of Brg1 and the phenotype of brg1 zebrafish show that Brg1 is critical for specific aspects of cardiac gene expression. As Brg1 +/− mice are underrepresented after birth [13] , we hypothesized that the partially penetrant lethality in Brg1 +/− mice might be due to CHDs. We found that 50% of Brg1 +/− mice died before 3 weeks of age (compared with 0% in WT controls), and in neonatal mice ( n =10) we found CHDs such as dilated hearts (5/10), muscular ventricular septal defects (2/10) and incomplete closure of the atrial septum (4/10), a condition known as patent foramen ovale ( Fig. 4a ). Specific heterozygous deletion of Brg1 in ventricular myocytes (with Nkx2.5::Cre ) and cardiac precursors (with Mef2cAHF::Cre [26] ) also led to CHDs, indicating that these are not due to nonspecific effects of loss of Brg1 outside the heart ( Supplementary Fig. S4 ). The lack of severe defects in Nkx2.5::Cre ; Brg1 fl /+ mice (in which heterozygous loss of Brg1 is only in ventricular myocytes) indicate that the defects in Brg1 +/− mice are likely to result from combined defects in multiple cardiac cell types. Brg1 +/− mice that survived the neonatal period had structurally normal hearts, but we also identified specific abnormalities in heart function in adult Brg1 +/− mice, as determined by high-frequency ultrasound and electrical function ( Fig. 4b–d ). Haemodynamic anomalies consisted of predominantly impaired cardiac relaxation, as determined primarily by a decrease in E-wave amplitude ( Fig. 4b,d ). Defects in cardiac electrical function were also found in surviving Brg1 +/− mice by telemetry electrocardiogram (ECG), which included atrioventricular block, mild prolongation of the QRS complex (indicative of slowed conduction) and occasional sinus node dysfunction (resulting in an irregular heart beat; Fig. 4b–d ). We conclude that Brg1 haploinsufficiency predisposes mice to CHDs and abnormal heart function. This important result identifies a dosage requirement for BAF complexes in specific aspects of cardiac morphogenesis and functional maturation, and suggests a potential mechanistic link to disease-causing mutations in human CHD. 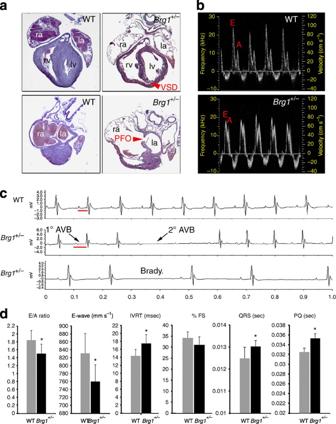Figure 4: CHDs inBrg1heterozygous null mice. (a) Histology of postnatal day 0 WT (left panels) andBrg1+/−hearts (right panels), showing dilated chambers, muscular ventricular septal defect (VSD) and patent foramen ovale (PFO) inBrg1+/−hearts. Top and bottom panels are planes of section of the same heart at the level of the outflow tract (top panels) and at the level of the atrial septum (bottom panels). Original magnification: ×50. (b) Doppler waveforms of flow at the mitral valve of adult WT andBrg1+/−mice, showing altered E and A wave amplitudes inBrg1+/−mice. (c) ECG telemetry in WT andBrg1+/−mice, showing prolonged PQ interval, sinus pause and second-degree atrioventricular block inBrg1+/−mice. (d) Quantitation of selected parameter in WT (grey bars) andBrg1+/−(black bars) mice. Units of measure are indicated in parentheses next to the graphed metric title. Data are mean±s.d.;n=5; *P<0.05. la, left atrium; lv, left ventricle; ra, right atrium; rv, right ventricle. Figure 4: CHDs in Brg1 heterozygous null mice. ( a ) Histology of postnatal day 0 WT (left panels) and Brg1 +/− hearts (right panels), showing dilated chambers, muscular ventricular septal defect (VSD) and patent foramen ovale (PFO) in Brg1 +/− hearts. Top and bottom panels are planes of section of the same heart at the level of the outflow tract (top panels) and at the level of the atrial septum (bottom panels). Original magnification: ×50. ( b ) Doppler waveforms of flow at the mitral valve of adult WT and Brg1 +/− mice, showing altered E and A wave amplitudes in Brg1 +/− mice. ( c ) ECG telemetry in WT and Brg1 +/− mice, showing prolonged PQ interval, sinus pause and second-degree atrioventricular block in Brg1 +/− mice. ( d ) Quantitation of selected parameter in WT (grey bars) and Brg1 +/− (black bars) mice. Units of measure are indicated in parentheses next to the graphed metric title. Data are mean±s.d. ; n =5; * P <0.05. la, left atrium; lv, left ventricle; ra, right atrium; rv, right ventricle. Full size image Brg1 genetically interacts with transcription factor genes The morphological and physiological heart defects in Brg1 +/− mice are reminiscent of those in Tbx5 haploinsufficient mice [4] , [27] , [28] . We hypothesized that Brg1 might be a critical determinant of the dosage sensitivity of Tbx5 . To look for a genetic interaction between Tbx5 and Brg1 , we generated mice heterozygous for both Tbx5 and Brg1 ( Brg1 +/− ; Tbx5 del/+ mice). Compared with Brg1 +/− or Tbx5 del/+ mice, which had normal heart morphologies at E12.5, all Brg1 +/− ; Tbx5 del/+ mice ( n =6) had severe defects in heart formation at this stage, including hypoplastic left ventricle and dilated atria ( Fig. 5a,b ). Although Brg1 +/− ; Tbx5 del/+ hearts appeared relatively normal at E11.5, this genetic interaction was evident at the level of Nppa gene expression at E9.5, which was expressed at normal levels in Brg1 +/− mice, at slightly reduced levels in Tbx5 del/+ mice, but was undetectable in Brg1 +/− ; Tbx5 del/+ mice ( Fig. 5a ). Trivial explanations might be that, in Brg1 +/− ; Tbx5 del/+ mice, the expression of Tbx5 is much lower than in Tbx5 del/+ or Brg1 +/− mice or that expression of its interacting partners ( Nkx2–5 , Gata4 ) is lower, predisposing the mice to more severe CHDs; this mechanism was discounted by quantitative reverse transcription-PCR and microarray analysis that showed similar levels of Tbx5 , Nkx2–5 and Gata4 messenger RNA (mRNA) in Brg1 +/− and Brg1 +/− ; Tbx5 del/+ hearts at E11.5 ( Supplementary Fig. S5 and Supplementary Data 1 ). 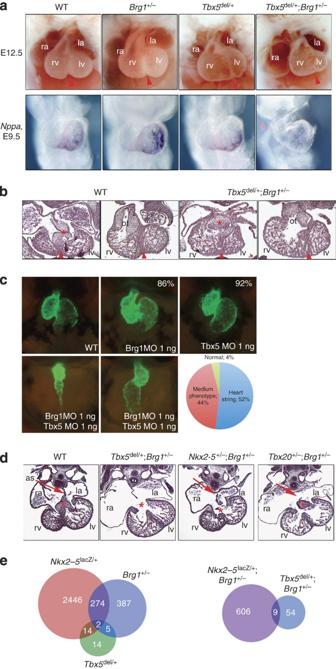Figure 5: Genetic interactions betweenBrg1and cardiac transcription factor genes. (a)Brg1andTbx5genetically interact. The top row shows an external view of hearts from E12.5 WT,Brg1+/−,Tbx5del/+andBrg1+/−;Tbx5del/+embryos; the bottom row shows expression ofNppaat E9.5 for the same genotypes. Original magnification: ×50. (b) Histology of E11.5 WT andBrg1+/−;Tbx5del/+embryos.Brg1+/−orTbx5del/+embryos are indistinguishable from WT. Asterisk indicates atrioventricular cushion and arrowhead indicates interventricular septum. Original magnification: ×100. (c)Brg1andTbx5interactions in zebrafish. Tg(cmlc2:eGFPtwu34) control (WT) or MO-injected embryos are shown in ventral–anterior views at 72 hpf. Brg1MO: MO directed againstBrg1; Tbx5MO: MO directed againstTbx5. All MOs were injected at 1 ng. Percentages in the Brg1MO and Tbx5MO show the percentage of normal hearts. The graph shows the percentage of phenotypes observed in double knockdown experiments (n=74, 91 and 126 forbrg1,tbx5andbrg1+tbx5morpholino injections, respectively). Original magnification: ×400. (d)Brg1genetically interacts withTbx5,Nkx2–5andTbx20. Histology of E12.5 hearts shows specific defects inBrg1+/−;Tbx5del/+,Brg1+/−;Nkx2–5+/−andBrg1+/−;Tbx20+/−embryos, compared with WT.Nkx2–5+/−andTbx20+/−hearts are structurally identical to WT hearts. Asterisk indicates atrioventricular cushion and arrow indicates atrial septum (as). Original magnification: ×100. (e) Summary of microarray analysis performed on E11.5 hearts of the indicated genotypes. Venn diagrams show the number of altered transcripts for each genotype, using a statistical cutoff ofP<0.01 and fold change >0.3. la, left atrium; lv, left ventricle; ot, outflow tract; ra, right atrium; rv, right ventricle. Figure 5: Genetic interactions between Brg1 and cardiac transcription factor genes. ( a ) Brg1 and Tbx5 genetically interact. The top row shows an external view of hearts from E12.5 WT, Brg1 +/− , Tbx5 del /+ and Brg1 +/− ; Tbx5 del /+ embryos; the bottom row shows expression of Nppa at E9.5 for the same genotypes. Original magnification: ×50. ( b ) Histology of E11.5 WT and Brg1 +/− ; Tbx5 del /+ embryos. Brg1 +/− or Tbx5 del /+ embryos are indistinguishable from WT. Asterisk indicates atrioventricular cushion and arrowhead indicates interventricular septum. Original magnification: ×100. ( c ) Brg1 and Tbx5 interactions in zebrafish. Tg( cmlc2:eGFP twu34 ) control (WT) or MO-injected embryos are shown in ventral–anterior views at 72 hpf. Brg1MO: MO directed against Brg1 ; Tbx5MO: MO directed against Tbx5 . All MOs were injected at 1 ng. Percentages in the Brg1MO and Tbx5MO show the percentage of normal hearts. The graph shows the percentage of phenotypes observed in double knockdown experiments ( n =74, 91 and 126 for brg1 , tbx5 and brg1 + tbx5 morpholino injections, respectively). Original magnification: ×400. ( d ) Brg1 genetically interacts with Tbx5 , Nkx2–5 and Tbx20 . Histology of E12.5 hearts shows specific defects in Brg1 +/− ; Tbx5 del /+ , Brg1 +/− ; Nkx2–5 +/− and Brg1 +/− ; Tbx20 +/− embryos, compared with WT. Nkx2–5 +/− and Tbx20 +/− hearts are structurally identical to WT hearts. Asterisk indicates atrioventricular cushion and arrow indicates atrial septum (as). Original magnification: ×100. ( e ) Summary of microarray analysis performed on E11.5 hearts of the indicated genotypes. Venn diagrams show the number of altered transcripts for each genotype, using a statistical cutoff of P <0.01 and fold change >0.3. la, left atrium; lv, left ventricle; ot, outflow tract; ra, right atrium; rv, right ventricle. Full size image In zebrafish, mutation of tbx5 in the heartstrings mutant [29] leads to defects in heart looping and progressive deterioration of the heart. The similarity between tbx5 and brg1 mutants in the fish raised the possibility that genetic interactions between these two genes may exist also in zebrafish. We performed double knockdown of brg1 and tbx5 via MOs. When 1 ng brg1 or tbx5 morpholino was injected, the heart developed normally in all cases ( Fig. 5c ). In contrast, co-injection of brg1 and tbx5 morpholino (1 ng each) resulted in 52% of embryos displaying a severe heartstrings -like phenotype and 44% of embryos having a milder unlooped, tube-like heart phenotype ( n =120; Fig. 5c ), demonstrating a clear and conserved genetic interaction between brg1 and tbx5 . We utilized the variable dose dependency of other critical cardiac transcription factors in the mouse to test further genetic interactions with Brg1 . Although Tbx5 haploinsuffiency in the mouse mimics CHDs in humans [4] , Nkx2–5 heterozygous mice display only very mild aspects of CHDs caused by human NKX2–5 mutations [30] , [31] , and Tbx20 haploinsufficiency does not result in any detectable heart defects [32] . We generated compound heterozygous mice for Brg1 and for either Tbx5 , Nkx2–5 or Tbx20 ; all mouse mutations are loss-of-function alleles with no known dominant activity. In all three cases, dramatic and specific defects in heart formation were observed in all compound heterozygous mice ( n =4–8) at E12.5 ( Fig. 5d ), and no compound heterozygous mice survived past E14.5. Defects included severe loss of cardiac cushion formation ( Tbx5 +/− ; Brg1 +/− and Brg1 +/− ; Nkx2–5 +/− ), thinned atrial walls ( Tbx5 +/− ; Brg1 +/− , Tbx20 +/− ; Brg1 +/− ), hypoplastic ventricles ( Tbx5 +/− ; Brg1 +/− , Nkx2–5 +/− ; Brg1 +/− ) and thinned ventricular walls ( Nkx2–5 +/− ; Brg1 +/− , Tbx20 +/− ; Brg1 +/− ). gata5 mutant fishes also have heart defects [33] , and mouse Gata4, the functional homologue of zebrafish gata5, interacts with BAF complexes [7] , [8] ; we also observed an interaction of brg1 and gata5 low-dose MOs, supporting a more general importance of dose-dependent interactions between Brg1 and cardiac transcription factors ( Supplementary Fig. S2 ). These strong genetic interactions between Brg1 and cardiac transcription factor genes in mouse and zebrafish demonstrate a finely regulated interdependency between cardiac DNA-binding transcription factors and BAF chromatin remodelling complexes. Programmes regulated by Brg1 and cardiac transcription factors The genetic interaction between Brg1 and cardiac transcription factor genes could be a result of a genetic programme common to all transcription factors that is sensitive to Brg1 levels or, alternatively, Brg1 may potentiate each transcription factor's specific genetic programme. To address this question, we performed transcriptional profiling of E11.5 hearts from mice heterozygous for deletions of Brg1 , Tbx5 or Nkx2–5 , and mice that were compound heterozygotes for Brg1 and each transcription factor gene. We observed varying degrees of overlap between the sets of genes that were altered by decreased dosages of Brg1 , Tbx5 and Nkx2–5 , indicating some specificity to the programmes that are regulated by these factors ( Fig. 5e and Supplemental Data 1 , and quantitative RT-PCR (QRT-PCR) validation in Supplementary Fig. S5 ). Clustering analysis defined specific groups of genetic interactions ( Fig. 6a,b ), indicating considerable complexity to the genetic interactions between Nkx2–5 or Tbx5 and Brg1 . For example, some genes were altered mostly in compound heterozygous hearts (clusters a, m, g, t). These genes are more resistant to an imbalance between Brg1 and the DNA-binding factors, but still rely on the balance of Brg1 and Tbx5 or Nkx2–5 for their normal regulation. Imbalance in the expression of these sets of genes is likely to be key for the compound heterozygous phenotype observed between Brg1 and Tbx5 or Nkx2–5 . 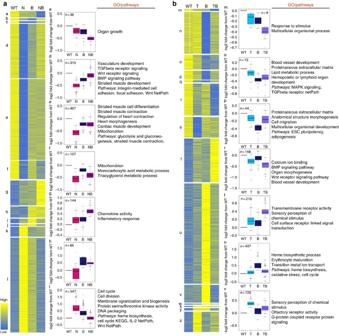Figure 6: Clustering analysis of altered gene expression. (a) Clustering analysis of altered transcripts fromNkx2–5+/−(N),Brg1+/−(B) and compound heterozygotes,Nkx2–5+/−;Brg1+/−(NB) E11.5 hearts. Heart maps for all statistically significant clusters indicate the average value for each group. All biological replicates within groups were included in cluster analyses; figures were made by taking the mean for each group. Box plots for a selection of clusters show the median (middle line), third and first quartile (top and bottom (hinges) of the boxes); the 'whiskers' extend 1.5× the length of the box, with other points (outliers) plotted as circles. Statistically significantly overrepresented Gene Ontology (GO) categories (adjustedP<0.01) are shown. Genotypes are shown on thexaxis;yaxis shows log 2 fold change from WT. (b) Clustering analysis as in B, but for transcripts fromTbx5del/+(T),Brg1+/−(B) and compound heterozygotes,Tbx5del/+;Brg1+/−(TB) E11.5 hearts. Figure 6: Clustering analysis of altered gene expression. ( a ) Clustering analysis of altered transcripts from Nkx2–5 +/− (N), Brg1 +/− (B) and compound heterozygotes, Nkx2–5 +/− ; Brg1 +/− (NB) E11.5 hearts. Heart maps for all statistically significant clusters indicate the average value for each group. All biological replicates within groups were included in cluster analyses; figures were made by taking the mean for each group. Box plots for a selection of clusters show the median (middle line), third and first quartile (top and bottom (hinges) of the boxes); the 'whiskers' extend 1.5× the length of the box, with other points (outliers) plotted as circles. Statistically significantly overrepresented Gene Ontology (GO) categories (adjusted P <0.01) are shown. Genotypes are shown on the x axis; y axis shows log 2 fold change from WT. ( b ) Clustering analysis as in B, but for transcripts from Tbx5 del/+ (T), Brg1 +/− (B) and compound heterozygotes, Tbx5 del/+ ; Brg1 +/− (TB) E11.5 hearts. Full size image Perhaps more surprisingly, many genes that were altered in single heterozygous ( Nkx2–5 lacZ/+ , Brg1 +/− or Tbx5 del/+ ) hearts compared with WT hearts were not significantly altered in compound heterozygous ( Nkx2–5 lacZ/+ ; Brg1 +/− or Tbx5 del/+ ; Brg1 +/− ) hearts (clusters d, e, l, n, o and u in Fig. 6a,b ). One possible interpretation of this striking interaction is that the relative levels of Nkx2–5 (or Tbx5) and Brg1 need to be maintained for normal expression of this set of genes, and that loss of one allele of either Nkx2–5 or Brg1 in single heterozygotes upsets this balance, leading to an allelic ratio of 2:1 or 1:2; however, in Nkx2–5 lacZ/+ ; Brg1 +/− hearts the balance is restored (a 1:1 allelic ratio). This implies that the relative levels between the DNA-binding factors (Tbx5 and Nkx2–5) and Brg1 is critical for a large set of genes. The types of genes identified in the transcriptional profiling assays were from a wide range of functional classes, as exemplified from statistical exploration of Gene Ontology classifications that revealed broad classes of transcripts enriched in specific clusters ( Fig. 6 ). Several genes important for heart development were identified in the different clusters of differentially regulated genes, including several previously identified as altered in Nkx2–5 - or Tbx5 -deficient hearts [31] , [34] , [35] . One particular novel set of transcripts was of interest: in Nkx2–5 lacZ/+ and Brg1 +/− hearts, we measured a clear increase in expression of several genes associated with the haematopoietic programme, including key regulators of this programme such as Gata1 , Klf1 and Tal1 . This implies that Nkx2–5/Brg1 suppresses haematopoietic differentiation in the embryonic heart. It is difficult to precisely link the contribution of the different genetic programmes regulated by individual factor dosage and combinatorial dosage to the heart defects in each genetic modification, especially with only one snapshot in developmental time. Furthermore, many of the affected transcripts are likely to be due to indirect effects. However, it is clear that overlapping programmes are sensitive to the dosage of Brg1 and the cardiac transcription factor genes. Reduced promoter occupancy by Brg1 in mutant hearts Genetic interactions between Brg1 and cardiac transcription factors may reflect a direct physical interaction that is sensitive to the dosage of each factor, in one or multiple cell types, as well as interactions between various cell types in which one factor is haploinsufficient, and another cell type in which the interacting factor is haploinsufficient. To address the former possibility, we performed chromatin immunoprecipitation (ChIP) for Brg1 on E9.5 hearts from WT, Tbx5 del/+ , Brg1 +/− and Tbx5 del/+ ; Brg1 +/− embryos at the cardiomyocyte-specific Nppa and Gja5 promoters ( Fig. 7a ). We found that at the Nppa gene, Brg1 occupancy was reduced in Brg1 +/− hearts, consistent with a limiting amount of Brg1, and that at both Nppa and Gja5 , Brg1 occupancy was reduced in Tbx5 del/+ hearts, indicating that reduced levels of Tbx5 directly result in reduced occupancy of Brg1 ( Fig. 7b ). Brg1 occupancy on both promoters was further reduced in Tbx5 del/+ ; Brg1 +/− embryos, suggesting that the interdependency of Tbx5 and Brg1 is partly compensated by interactions with other factors, perhaps other transcription factors that can interact with BAF complexes. These results provide a mechanism for some of the dosage-related relationships between Tbx5 and Brg1 on Tbx5 target genes, and support the notion that at least some of the effects of the genetic interaction between Tbx5 and Brg1 reflect cell-autonomous direct interactions. 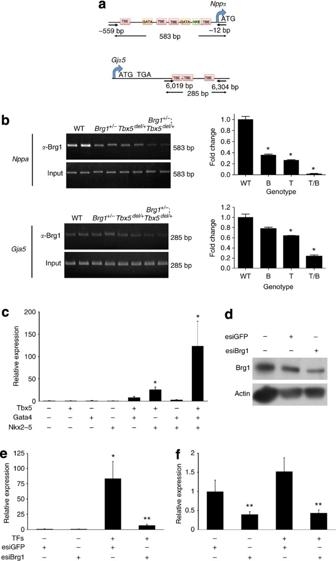Figure 7: Direct interactions between Brg1 and cardiac transcription factors. (a) Diagram indicating the location of primer pairs for amplification of immunoprecipitated chromatin-associated DNA forNppaandGja5. Locations of conserved T-box-binding elements (TBE), GATA factor-binding sites (GATA) and Nkx2–5-binding sites (NKE) are shown. ATG: start codon; TGA: translational stop codon. Nucleotide positions shown are relative to start codon. (b) ChIP of Brg1 at theNppaorGja5promoters from E9.5 hearts of the indicated genotypes. On the left are EtBr-stained gels showing amplification, and quantitation by QPCR is shown in the graphs on the right. Data are mean±s.e.;n=3; *P<0.05. (c) Quantitation ofNppamRNA in NIH3T3 fibroblasts transfected with combinations of Tbx5, Nkx2–5 and Gata4. Data are mean±s.e.;n=3; *P<0.05 versus mock transfection. (d) Western blot to measure reduction of Brg1 protein levels by anti-Brg1 esiRNAs. Actin is a loading control. (e) Quantitation ofNppamRNA in NIH3T3 fibroblasts transfected with Tbx5, Nkx2–5 and Gata4, with or without esiRNAs targeting Brg1, or control esiRNAs. TFs=Tbx5, Gata4 and Nkx2–5. Data are mean±s.e.;n=3; *P<0.05 versus mock transfection; **P<0.05 esiBrg1+versus esiBrg1−. (f) Brg1 mRNA levels in the same samples as inc. Data are mean±s.e.;n=3; **P<0.05 esiBrg1+versus esiBrg1−. Figure 7: Direct interactions between Brg1 and cardiac transcription factors. ( a ) Diagram indicating the location of primer pairs for amplification of immunoprecipitated chromatin-associated DNA for Nppa and Gja5 . Locations of conserved T-box-binding elements (TBE), GATA factor-binding sites (GATA) and Nkx2–5-binding sites (NKE) are shown. ATG: start codon; TGA: translational stop codon. Nucleotide positions shown are relative to start codon. ( b ) ChIP of Brg1 at the Nppa or Gja5 promoters from E9.5 hearts of the indicated genotypes. On the left are EtBr-stained gels showing amplification, and quantitation by QPCR is shown in the graphs on the right. Data are mean±s.e. ; n =3; * P <0.05. ( c ) Quantitation of Nppa mRNA in NIH3T3 fibroblasts transfected with combinations of Tbx5, Nkx2–5 and Gata4. Data are mean±s.e. ; n =3; * P <0.05 versus mock transfection. ( d ) Western blot to measure reduction of Brg1 protein levels by anti-Brg1 esiRNAs. Actin is a loading control. ( e ) Quantitation of Nppa mRNA in NIH3T3 fibroblasts transfected with Tbx5, Nkx2–5 and Gata4, with or without esiRNAs targeting Brg1, or control esiRNAs. TFs=Tbx5, Gata4 and Nkx2–5. Data are mean±s.e. ; n =3; * P <0.05 versus mock transfection; ** P <0.05 esiBrg1 + versus esiBrg1 − . ( f ) Brg1 mRNA levels in the same samples as in c . Data are mean±s.e. ; n =3; ** P <0.05 esiBrg1 + versus esiBrg1 − . Full size image Brg1-dependent transcriptional activation in vitro We investigated whether transcriptional activation of cardiac genes directly requires the function of Brg1. We previously showed that Tbx5, Nkx2–5, Gata4 and the BAF complex subunit Baf60c can activate cardiac gene expression in non-cardiac mesoderm [8] . We found that co-transfection of NIH3T3 fibroblasts with Tbx5, Nkx2–5 and Gata4 expression constructs could robustly induce de novo the cardiac-specific gene Nppa , a marker of differentiated cardiomyocytes, the promoter of which is well characterized as a target of these transcription factors ( Fig. 7c ) (refs 4 , 36 ). As Baf60c is expressed in NIH3T3 fibroblasts, exogenous Baf60c did not enhance the effect (data not shown). Other cardiac genes examined were not induced by this combination of factors. To determine the requirement for Brg1 in the de novo activation of Nppa , we depleted Brg1 with endoribonuclease prepared small interfering RNAs (esiRNAs) [37] . esiRNAs directed against Brg1 resulted in an ∼ 50% decrease in Brg1 protein level ( Fig. 7d ). Decreased levels of Brg1 completely prevented Nppa activation by cardiac transcription factors ( Fig. 7e,f ), suggesting that this transcriptional activation is dependent on limiting amounts of functional Brg1-containing BAF complexes. We demonstrated a critical, conserved and dosage-sensitive role for the BAF chromatin remodelling complex ATPase Brg1 in vertebrate heart development. Our results further show an important interdependency between BAF complexes and disease-related cardiac transcription factors, which suggests a mechanism for CHDs caused by mutations in these transcription factor genes and implications for multigenic inheritance of CHDs. In mouse and zebrafish, Brg1 is required for important and specific aspects of heart development. In particular, chamber morphogenesis is disrupted in both mice and fish lacking Brg1, and proliferation of cardiac progenitors is reduced. A key subset of cardiac genes was affected by the loss of Brg1 , consistent with specific roles for BAF complexes in differentiation of other cell types [9] , [14] , [19] , [38] , [39] , [40] , [41] , [42] . In many of these cases, Brg1 is required for differentiation after specification. Our results support a clear role for Brg1 in cardiac differentiation. As the function of Gata4, Nkx2–5 and Tbx5 relies on BAF complexes, in part via Baf60c [7] , [8] , loss of Brg1 likely affects target genes primarily by reducing the activation potential of cardiac transcription factors. Loss of brg1 in zebrafish demonstrates a strikingly conserved role for BAF complexes in vertebrate cardiac development. The morphogenetic and gene expression defects in brg1 mutant fish closely resemble that seen in mice lacking Brg1 , suggesting that the gene networks regulated by BAF complexes are well conserved in vertebrate evolution. Notably, mice heterozygous for a deletion of Brg1 have heart defects. This important finding indicates that Brg1 is haploinsufficient in the heart. Haploinsufficiency of Brg1 has been reported in the brain [13] and immune system [43] , indicating that certain cell types are sensitive to the dosage of Brg1 . The important dose dependency of Brg1 function in cardiogenesis shows that, as for DNA-binding transcription factors, normal formation of the heart relies on precise levels of functional BAF complexes. Furthermore, the genetic interaction between Brg1 and several cardiac transcription factor genes shows that transcription factor function is intimately linked to levels of Brg1. The resulting CHDs are likely to reflect these interactions in multiple cell types. Our promoter occupancy data indicate that, for at least a portion of co-regulated genes, a direct cell-autonomous dosage-related interaction exists. Specific genetic programmes are sensitive to the dosage of each transcription factor, and there is considerable complexity in the genomic regulation of gene expression by Brg1 and cardiac transcription factors. In some cases, a clear interrelationship exists between the dosage effects of either factor, resulting in a more profound effect in embryos haploinsufficient for Brg1 and Nkx2–5 or Tbx5 . In other words, diminution of levels of one factor will reduce that factor's chance of interaction with BAF complexes, and this can be accentuated when Brg1 levels are also lower. Our molecular data support a model ( Fig. 8 , model a) for direct interactions between Brg1 and cardiac transcription factors, and imply that reduced recruitment of BAF complexes may be a significant molecular mechanism underlying transcription factor haploinsufficiency in congenital heart disease. 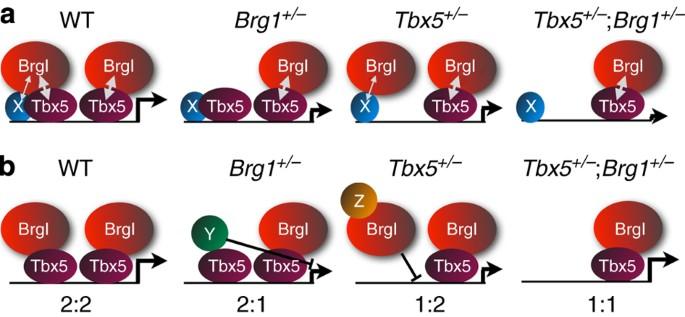Figure 8: Models for the interaction between DNA-binding transcription factors and Brg1. Two models for the interaction between DNA-binding transcription factors and Brg1. Model (a) is based on the dosage-sensitive interrelationship between DNA-binding transcription factors (represented by Tbx5) and Brg1. InBrg1+/−hearts, some Tbx5-binding events are not accompanied by concomitant Brg1 binding, resulting in decreased gene expression. InTbx5+/−hearts, Brg1 can only interact with one of two potential Tbx5-binding events, but may still interact more weakly with other DNA-binding transcription factors (X). InTbx5+/−;Brg1+/−hearts, all quantitative interactions are impaired, leading to further reduction in target gene expression. Model (b) is based on the normalization of gene expression inTbx5+/−;Brg1+/−andNkx2-5+/−;Brg1+/−hearts, and is based on the allelic balance between the two genes. InBrg1+/−hearts, the ratio of Tbx5 to Brg1 alleles is now 2:1, which allows some Tbx5-binding events to interact with other factors, including a hypothetical repressor protein (Y). InTbx5+/−hearts, the ratio of Tbx5 to Brg1 alleles is now 1:2, which allows some Brg1-binding events to interact with other factors, including a hypothetical repressor or sequestrating protein (Z). InTbx5+/−;Brg1+/−hearts, the balance is restored to 1:1, eliminating the potential for other interactions. Figure 8: Models for the interaction between DNA-binding transcription factors and Brg1. Two models for the interaction between DNA-binding transcription factors and Brg1. Model ( a ) is based on the dosage-sensitive interrelationship between DNA-binding transcription factors (represented by Tbx5) and Brg1. In Brg1 +/− hearts, some Tbx5-binding events are not accompanied by concomitant Brg1 binding, resulting in decreased gene expression. In Tbx5 +/− hearts, Brg1 can only interact with one of two potential Tbx5-binding events, but may still interact more weakly with other DNA-binding transcription factors (X). In Tbx5 +/− ; Brg1 +/− hearts, all quantitative interactions are impaired, leading to further reduction in target gene expression. Model ( b ) is based on the normalization of gene expression in Tbx5 +/− ; Brg1 +/− and Nkx2-5 +/− ; Brg1 +/− hearts, and is based on the allelic balance between the two genes. In Brg1 +/− hearts, the ratio of Tbx5 to Brg1 alleles is now 2:1, which allows some Tbx5-binding events to interact with other factors, including a hypothetical repressor protein (Y). In Tbx5 +/− hearts, the ratio of Tbx5 to Brg1 alleles is now 1:2, which allows some Brg1-binding events to interact with other factors, including a hypothetical repressor or sequestrating protein (Z). In Tbx5 +/− ; Brg1 +/− hearts, the balance is restored to 1:1, eliminating the potential for other interactions. Full size image The observation that expression levels of several transcripts that are altered in heart heterozygous for a null allele of Nkx2–5 , Tbx5 or Brg1 are restored to normal or near-normal levels in Nkx2–5 lacz /+ ; Brg1 +/− or Tbx5 lacz /+ ; Brg1 +/− compound heterozygous hearts indicates that for some genes, the relative allelic balance of Nkx2–5 (or Tbx5 ) and Brg1 may be more important than their absolute levels. The mechanism underlying this dosage interdependence is not known, but may include increased potential for interaction with other proteins that would alter the functional output on target genes ( Fig. 8 , model b). Thus, haploinsufficiency of cardiac transcription factors in CHDs is predicted to result in an imbalance between transcription factors and BAF complexes, likely resulting in impaired transcriptional activation at loci sensitive to this balance. The reason for distinct dosage-sensitive responses from one group of genes to the next is not known, but perhaps the chromatin status of some genes requires different dosage-related interactions between BAF complexes and DNA-binding transcription factors. We cannot discern which specific group of genes, between those that respond more in the compound heterozygotes, those that return to WT levels in compound versus single heterozygotes, or combinations thereof, is responsible for the phenotypic output of transcription factor or Brg1 haploinsufficiency. It is likely that deregulation of many different genes in various functional classes would be responsible for the complex altered morphology and function that we observe. In conclusion, we demonstrated a critical requirement for Brg1 in the development of the vertebrate heart, and importantly showed that there exists a fine balance between Brg1 levels and those of cardiac transcription factors that have been implicated in human CHD. The genetic interactions between Brg1 and cardiac transcription factor genes predict that, in the developing heart, maintaining relative levels of BAF complexes and transcription factors is critical for the timely and precise activation of groups of genes during development. In human congenital heart disease, disruption of these dosage-sensitive interactions would predict the impaired activation of specific gene networks that are essential for specific aspects of cardiac morphogenesis and function. We propose that an imbalance in this relationship is a molecular basis underlying CHDs caused by mutations in cardiac transcription factors. Although such a finely regulated interrelationship is perhaps more prone to disruption, it confers significant advantages in the fine quantitative regulation of transcript levels, which is an essential component of complex morphogenesis. These results further underscore the potential for multigenic effects on dominant mutations, and suggest that polymorphisms in BAF complex subunit genes, including but not restricted to Brg1 , may modulate the penetration and phenotypic consequence of disease-causing mutations in transcription factor genes in human populations. Mouse strains and embryology The following mouse strains were used: Brg1 L2 /+ [14] , Nkx2–5::Cre [15] , Mef2cAHF::Cre [26] , Tbx5 del /+ [4] , Nkx2–5 lacZ /+ [35] , Tbx20 +/− [32] , Z/EG [44] and RYR [45] . Brg1 +/− mice were generated by crossing Brg1 L2/− mice with EIIa-Cre mice [46] . For all experimental analyses, at least three embryos per genotype were examined. All animal experiments were conducted following guidelines established and approved by the UCSF Institutional Animal Care and Use Committee, and in accordance with best practices outlined by the Canadian Council on Animal Care and licensed by Lab Animal Services at the Hospital for Sick Children. Analysis of protein and mRNA expression Immunostaining and in situ hybridization procedures were carried out by standard protocols. For immunostaining, cryosections were incubated with primary antisera against enhanced green fluorescent protein (EGFP; Abcam ab13970, 1:300) and with alpha-tropomyosin (CH1 monoclonal, Hybridoma bank, 1:50), followed by incubation with Alexa Fluor 488-coupled goat-anti-chicken immunoglobulin (Ig) G (Invitrogen A11039, 1:200) and Alexa Fluor 594-coupled goat anti-mouse IgG (Invitrogen A110320), and were mounted with Prolong gold with 4,6-diamidino-2-phenylindole (Invitrogen), to stain nuclei. In situ hybridization by whole mount or on 10 μm paraffin sections was performed using previously described protocols [47] . RNA probes were labelled with digoxigenin-labelled UTP, hybridized to samples and after washes were incubated with alkaline phosphatase-coupled anti-digoxigenin antisera (Roche); colorimetric detection was carried out by incubation with BM purple (Roche). Optical projection tomography (OPT) was performed as described [7] using embryos labelled for alpha-cardiac actin ( Actc ) by fluorescent in situ hybrization (using the TSA amplification system, Amersham). OPT images were acquired in the GFP channel for tissue autofluorescence, and in the red channel for Actc fluorescence. Three-dimensional reconstructions were analysed and rendered in Amira 4.0 (Visage Imaging). QRT-PCR was performed with Taqman probe sets ( Supplementary Table S1 ). Cardiac physiology Cardiac function was assessed by high-frequency ultrasound and telemetry ECG [4] , [27] . For ultrasound assessment of cardiac function, a high-frequency ultrasound imaging system (Vevo 660, VisualSonics) with a 30 MHz transducer was used for in vivo evaluation of cardiac morphology and function as previously described in detail [27] Mice were anaesthetized with isoflurane at 1.5% by face mask, and body temperature was maintained at ∼ 37 °C. An M-mode recording of the left ventricle was made in long-axis view and analysed for wall thickness and chamber dimension. Fractional shortening was also calculated as a measure of left ventricular systolic function. Mitral Doppler flow spectrum was recorded in apical four-chamber view, with the Doppler sample volume placed at the centre of mitral orifice and at the tip level of the valves for the highest velocities. The peak velocities of the early ventricular filling wave (E wave) and the late ventricular filling wave caused by atrial contraction (A wave) were measured, and their ratio was calculated. The left ventricular systolic and diastolic time intervals were also measured, including the isovolumic relaxation time, ventricular diastolic filling time, isovolumic contraction time and ventricular ejection time. All parameters were averaged for three cardiac cycles. For ECG telemetry, telemetry devices (DSI) were implanted subcutaneously dorsally under anaesthesia (sodium pentobarbital, 0.033 mg g −1 i.p. ), and the leads were placed in lead II conformation. Following a 72 h recovery period, mice housed in individual cages were placed on telemetry detection platforms and continuous ECG tracings were acquired for 24 h. ECGs were manually examined for arrhythmias. Ultrasound measurements and ECG intervals were calculated during periods of regular sinus rhythm. Zebrafish embryology and genetics The brg1 s481 allele was identified in a diploid ENU mutagenesis screen for mutations affecting endodermal organ morphogenesis [48] . A C-to-T base-pair change at position 754 in the brg1 (smarca4) coding sequence creates a premature STOP codon at amino acid 252. MOs targeting brg1 and p53 have been previously published and validated [20] , [21] . RNA in situ hybridization probes for myl7/cmlc2, nppa, bmp4, tbx2b and notch1b have been characterized [49] , [50] . For the ncx1h ( slc8a1a ) probe, a 560 bp PCR product amplified from cDNA was used as a template. For mosaic labelling of cardiomyocytes, embryos from Tg( cmlc2:eGFP twu34 ) +/+ in-crosses were injected at the one-cell stage with 10 pg of pBISceI-cmlc2:dsRed plasmid DNA with I SceI enzyme (NEB) in I SceI buffer. For time-lapse analysis, Tg (cmlc2:eGFP) control embryos or morphants were mounted in agarose, and imaged at 28.5 °C using a 25× water objective. To count cardiomyocytes at various stages, we used the Tg( cmlc2:dsRedExp-nuc hsc4 ) line. Mounted embryos were imaged with a 40× water immersion lens. Sequential confocal images were taken with a standardized step size of 0.65 ìm in the z -direction. Quantification of myocardial cells, cell migration tracking and three-dimensional reconstructions of confocal stacks were carried out using Volocity (Improvision). Microarrays and statistical analysis Affymetrix mouse Gene ST 1.0 arrays were hybridized and scanned according to the manufacturer's recommendations. Raw intensities from CEL files were analysed using Affymetrix Power Tools (APT, version 1.10.1) to generate robust multiarray average [51] expression intensities on a log-2 scale for each probe set and various quality metrics. The probe intensities were background-corrected, quantile-normalized and summarized for each probe set using a robust fit of linear models. Linear models were fitted for each gene to estimate genotype effects and associated significance using the limma package [52] in R/Bioconductor. Because sample sizes are often small in microarray experiments, the eBayes function in limma computes s.e. that are moderated across all genes on the array. The interpretation of the moderated t-statistics is the same as an ordinary t-statistics. Nkx2–5 / Brg1 and Tbx5 / Brg1 experiments were analysed separately using 2×2 factorial models. Linear contrasts were used to extract comparisons of interest. P-values were adjusted for multiple testing by controlling for false-discovery rate using the Benjamini–Hochberg method [53] . Genes differentially expressed >1.3-fold with adjusted P <0.01 were considered significantly different between groups. QRT-PCR and ChIP data were analysed by analysis of variance, followed by post hoc Tukey's test; P <0.05 was considered significant. Pairwise comparisons were made using t -test; P <0.05 was considered significant. Clustering and pathway analysis Genes that were declared to be differently expressed were subjected to unsupervized cluster analysis with the R package HOPACH [54] . All biological replicates within groups were included in cluster analyses. Pearson's correlations between genes were used as the distance metric, and default settings were used for other parameters. Clusters with similar expression patterns between genotypes were collapsed for further analysis. GOElite ( www.genmapp.org/go_elite/go_elite.html / ) was used to identify overrepresented gene ontology terms and pathways among the sets of differentially expressed genes. All genes that were subjected to expression analysis were used as the 'denominator' gene list for detecting overrepresentation. Null distributions were derived by permutation ( n =2000). Significance was assessed using false-discovery rate-adjusted P -values. Cell culture and ChIP NIH/3T3 mouse embryonic fibroblasts were seeded in a 24-well format at 40,000 cells per well; 2 days after seeding, cells were transfected using Lipofectamine 2000 reagent (Invitrogen) with a combination of HA-Tbx5, myc-GATA4 and FLAG-Nkx2–5 overexpression plasmids (200 ng) or empty pcDNA3.1 − (600 ng total). esiRNAs were generated as described [37] ; briefly, regions of EGFP or Brg1 were amplified by PCR (using the following primers: eGFP_esi1 (forward): 5′-TAATACGACTCACTATAGGGCGTAAACGGCCACAAGTTCA-3′; eGFP_esi2 (reverse): 5′-TAATACGACTCACTATAGGGATGGGGGTGTTCTGCTGGTA-3′; Brg1 esiRNA (forward): 5′-GGGCGGGTGTGTCCCTGTACAACAACAACC-3′; Brg1 esiRNA (reverse): 5′-GGGCGGGTCTGCAGCTCTTGAAGATAGTGG-3′. Brg1 PCR products were further amplified with an adaptor primer containing T7 sequences (5′-TAATACGACTCACTATAGGGAGACCACGGGCGGGT-3′). EGFP and Brg1 products were then purified using a Qiagen PCR Clean Up kit and were in vitro transcribed using T7 RNA polymerase (Roche). Transcribed RNA was annealed to yield double stranded RNA. After purification (Roche; Quick Spin Columns), 10 μg of double stranded RNA was subjected to digestion using purified glutathione S -transferase (GST)-RNAse III fusion protein and purified by ethanol precipitation to generate pools of 21 bp esiRNAs. In knockdown experiments, 450 ng of either esiGFP or esiBrg1 was transfected. Relative expression was determined by quantitative PCR using TaqMan probes against Nppa and Brg1 ; expression was normalized to β-actin (probe-set details in Supplementary Table S1 ). Each reaction was performed in technical triplicate. ChIP was performed as previously described [8] , using chromatin isolated from E12.5 embryonic hearts, with anti-Brg1 antiserum (Upstate 07-478) or normal rabbit IgG (Santa Cruz 2027), using 1 μg of antiserum. PCR was performed using the following primers: Nppa-595F: 5′-TCTTTCACCTGACTGCTAACA-3′, Nppa-12R: 5′-AGCATCTCCCGTTTTTATAG-3′; Gja5-F1: 5′-ACGACTGTGGCAGCAGGTGTTCTGC-3′, Gja5-R1: 5′-AGAACCAGCAGGTGCCCTTTCCCCT-3′. Amplicons were 573 bp long for Nppa and 583 bp long for Gja5 . Quantification was performed using the same primers and SYBR green quantification. Accession codes: Microarray data have been deposited in GEO under the accession number GSE26191 . How to cite this article: Takeuchi, J. K. et al . Chromatin remodelling complex dosage modulates transcription factor function in heart development. Nat. Commun. 2:187 doi: 10.1038/ncomms1187 (2011).